Doublecortin-like kinase enhances dendritic remodelling and negatively regulates synapse maturation Dendritic morphogenesis and formation of synapses at appropriate dendritic locations are essential for the establishment of proper neuronal connectivity. Recent imaging studies provide evidence for stabilization of dynamic distal branches of dendrites by the addition of new synapses. However, molecules involved in both dendritic growth and suppression of synapse maturation remain to be identified. Here we report two distinct functions of doublecortin-like kinases, chimeric proteins containing both a microtubule-binding domain and a kinase domain in postmitotic neurons. First, doublecortin-like kinases localize to the distal dendrites and promote their growth by enhancing microtubule bundling. Second, doublecortin-like kinases suppress maturation of synapses through multiple pathways, including reduction of PSD-95 by the kinase domain and suppression of spine structural maturation by the microtubule-binding domain. Thus, doublecortin-like kinases are critical regulators of dendritic development by means of their specific targeting to the distal dendrites, and their local control of dendritic growth and synapse maturation. Dynamic reorganization of microtubules (MTs) is a key component of many aspects of neuronal development and functions, including migration, process outgrowth and synapse formation. MT-associated proteins (MAPs) regulate the dynamics and organization of MTs. In addition to classical neuronal MAPs, such as MAP2 and tau, recent genetic analyses of mutations associated with developmental brain disorders identified new classes of MAPs, which are important in regulation of neuronal precursor migration [1] . Doublecortin (DCX) was identified as one of the causative genes of lissencephaly (‘smooth brain’) [2] and has been shown to contain MT-binding modules distinct from classical MAPs [3] . DCX expression is predominant in migrating neuronal precursors and is rapidly downregulated in differentiated neurons [4] , [5] ; the restricted expression of DCX could therefore explain its specific function in precursor migration. These observations indicate important roles for DCX in regulation of MT-dependent cell motility. DCX has two close homologues in mice: DCX-like kinase 1 (DCLK1) and DCX-like kinase 2 (DCLK2) [6] , [7] . These genes are widely expressed in the nervous system and have been reported to show persistent expression in adult neurons. Although the N termini of DCLK1 and 2 encode a MT-binding domain with high homology to DCX, the C termini of DCLK1 and 2 are unique and encode a domain similar to Ca 2+ /calmodulin-dependent kinases (CaMKs). Persistent expression of DCLKs and their unique domain organization suggest specific regulatory roles of DCLKs in postmitotic neurons. Recent proteomic analyses of biochemically purified postsynaptic density (PSD) fractions identified DCLKs as candidate PSD components [8] , [9] . Direct interaction of DCLK1 with spinophilin, a postsynaptic actin-bundling protein [10] , can also be taken as supportive evidence for synaptic functions of DCLKs. However, there are few reports demonstrating roles of DCLKs in differentiated neurons. Here we report two distinct functions of DCLKs in differentiated neurons. First, DCLKs preferentially localize at the distal dendrites and promote growth of dendrites via their two DCX tandems in the N-terminal segment. Second, DCLKs suppress maturation of glutamatergic synapses through multiple pathways, including reduction of PSD-95 via the kinase domain and suppression of spine structural maturation via the MT-binding domain. We postulate that DCLKs are strategically localized to the distal dendrites to achieve enhancement of process outgrowth and suppression of synapse maturation, both of which are important in maintaining structural plasticity of dendrites. Presence of DCLK in dendritic and postsynaptic compartments DCLK1 gives rise to multiple transcripts, and three major splice variants exist in the brain ( Fig. 1a ): a full-length isoform (long form), a short isoform with a MT-binding domain (DCX-like; DCL) and another short isoform with a kinase domain (short form) [11] , [12] , [13] , [14] . Furthermore, two major splice variants of DCLK2 exist; both of these contain the DCX domain and the kinase domain [15] . We generated a polyclonal pan-DCLK-antibody by using the DCLK1 DCX domain as an antigen ( Supplementary Fig. S1 ). This region shows high homology between DCLK1 and DCLK2, and our antibody showed comparable reactivity with both DCLK1 (long form) and DCLK2. Western blotting with this antibody revealed immunoreactive bands of 85 kDa, corresponding to the size of DCLK1 (long form) and DCLK2 in extracts of the cerebrum, cerebellum and hippocampus ( Fig. 1b ). The additional immunoreactivity of 43 kDa was likely to correspond to DCL and disappeared in samples taken from DCLK1 −/− mice ( Supplementary Fig. S1C ). The level of DCL was much lower than the level of DCLK1 (long form) and DCLK2 in the postnatal brain. DCLK expression was highest at postnatal day 7 and gradually decreased in the cerebrum and cerebellum ( Fig. 1b ). In the hippocampus, DCLK expression peaked around postnatal day 14 and started to decline thereafter. The immunoblots also showed weak nonspecific bands of 70 kDa, which did not disappear in samples taken from DCLK1 −/− and DCLK2 −/− mice ( Supplementary Fig. S1C ). 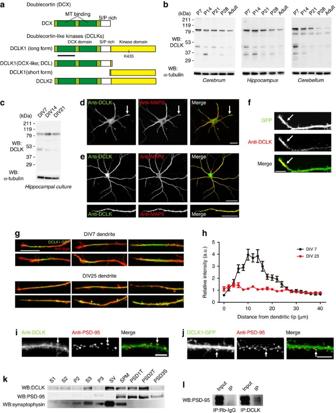Figure 1: Postnatal expression and subcellular localization of DCLKs. (a) Domain organizations of DCX, DCLK1 isoforms and DCLK2. A black line indicates the DCLK1 fragment used for antibody generation. S/P rich, serine/proline-rich domain. (b,c) Western blotting of DCLK protein. The immunoreactive bands of 85 kDa corresponding to the size of the full-length DCLK1 and DCLK2 proteins were detected in the extracts prepared from multiple brain regions (b) or dissociated hippocampal neurons at various days after plating (c). (d,e) Immunocytochemistry of dissociated hippocampal neurons at 7 DIV (d) and 24 DIV (e) using anti-DCLK and anti-MAP2 antibodies. DCLK proteins were preferentially concentrated in the distal part of dendrites at 7 DIV (arrows). (f) Immunocytochemistry of GFP-expressing hippocampal neurons with anti-DCLK antibody at 7 DIV. DCLK proteins were preferentially concentrated in the distal part of dendrites (arrows). (g) Transfection of DCLK1-GFP together with a lacZ reporter plasmid and subsequent immunocytochemistry with an anti-β-galactosidase antibody. (h) Relative intensity of DCLK1-GFP and anti-β-galactosidase immunoreactive signals at 7 DIV and 25 DIV. (DIV 7:n=13 cells, DIV 25:n=15 cells.) (i,j) Presence of DCLK immunoreactivity and DCLK1-GFP fluorescence in PSD-95-positive spines (arrows). (k) Presence of DCLK immunoreactivity in PSD-1T and PSD-2T fractions, which contain purified PSDs (P2: crude synaptosomal pellet, S3: crude synaptic vesicle fraction, P3: lysed synaptosomal membrane fraction, SV: synaptic vesicle fraction, SPM: synaptic plasma membrane fraction, PSD-1T,PSD-2T: purified PSD fractions, PSD3S: PSD fraction after sarkosyl treatment). (l) Immunoprecipitation of PSD-95 by anti-DCLK antibody in extracts from the adult brain (rabbit IgG (Rb-IgG) as a control antibody of immunoprecipitation). All numeric data are given as mean±s.e.m. Bar, 20 μm ford, 50 and 20 μm fore, 10 μm forfandgand 5 μm foriandj. Figure 1: Postnatal expression and subcellular localization of DCLKs. ( a ) Domain organizations of DCX, DCLK1 isoforms and DCLK2. A black line indicates the DCLK1 fragment used for antibody generation. S/P rich, serine/proline-rich domain. ( b , c ) Western blotting of DCLK protein. The immunoreactive bands of 85 kDa corresponding to the size of the full-length DCLK1 and DCLK2 proteins were detected in the extracts prepared from multiple brain regions ( b ) or dissociated hippocampal neurons at various days after plating ( c ). ( d , e ) Immunocytochemistry of dissociated hippocampal neurons at 7 DIV ( d ) and 24 DIV ( e ) using anti-DCLK and anti-MAP2 antibodies. DCLK proteins were preferentially concentrated in the distal part of dendrites at 7 DIV (arrows). ( f ) Immunocytochemistry of GFP-expressing hippocampal neurons with anti-DCLK antibody at 7 DIV. DCLK proteins were preferentially concentrated in the distal part of dendrites (arrows). ( g ) Transfection of DCLK1-GFP together with a lacZ reporter plasmid and subsequent immunocytochemistry with an anti-β-galactosidase antibody. ( h ) Relative intensity of DCLK1-GFP and anti-β-galactosidase immunoreactive signals at 7 DIV and 25 DIV. (DIV 7: n =13 cells, DIV 25: n =15 cells.) ( i , j ) Presence of DCLK immunoreactivity and DCLK1-GFP fluorescence in PSD-95-positive spines (arrows). ( k ) Presence of DCLK immunoreactivity in PSD-1T and PSD-2T fractions, which contain purified PSDs (P2: crude synaptosomal pellet, S3: crude synaptic vesicle fraction, P3: lysed synaptosomal membrane fraction, SV: synaptic vesicle fraction, SPM: synaptic plasma membrane fraction, PSD-1T,PSD-2T: purified PSD fractions, PSD3S: PSD fraction after sarkosyl treatment). ( l ) Immunoprecipitation of PSD-95 by anti-DCLK antibody in extracts from the adult brain (rabbit IgG (Rb-IgG) as a control antibody of immunoprecipitation). All numeric data are given as mean±s.e.m. Bar, 20 μm for d , 50 and 20 μm for e , 10 μm for f and g and 5 μm for i and j . Full size image DCLK expression in cultured hippocampal neurons was also maintained throughout the culture period with the peak of expression at 14 days in vitro (DIV) ( Fig. 1c ). Because our hippocampal primary culture contains few glial cells, this result indicates continual expression of DCLK1 (long form) or DCLK2 in postmitotic neurons. We could also detect DCLK proteins in cortical and hippocampal pyramidal neurons by immunohistochemistry of adult brain sections ( Supplementary Fig. S2 ). Specificity of our antibody was confirmed by significant reduction of immunoreactivity in primary neurons transfected with RNA interference (RNAi) constructs for both DCLK1 and DCLK2 (Fig. 3a). From these results, we concluded that DCLK protein expression is maintained in postnatal neurons, both in the cerebral cortex and hippocampus. DCLK proteins were enriched in dendrites of cultured hippocampal neurons at both 7 DIV and 24 DIV ( Fig. 1d ). Although DCLKs and a dendritic marker, MAP2, showed similar uniform distribution along dendrites at 24 DIV ( Fig. 1e ), DCLK proteins were enriched in the distal segments of dendrites at 7 DIV ( Fig. 1d , arrows). Preferential enrichment of DCLK immunoreactivity and DCLK1-green fluorescent protein (GFP) fluorescence was further confirmed by comparison with volume markers (GFP or β-galactosidase immunoreactivity; Fig. 1f ). Quantitative analysis of the relative intensity of DCLK1-GFP against anti-β-galactosidase fluorescence along the distal dendritic segments showed a clear peak only at 7 DIV ( Fig. 1h ). Previous studies revealed the presence of DCLK in biochemically purified PSD fraction [8] , [9] , [16] . Double labelling of cultured hippocampal neurons with both anti-DCLK and anti-PSD-95, a major postsynaptic scaffolding protein, revealed the presence of DCLKs in PSD-95-positive dendritic spines ( Fig. 1i ). Exogenously expressed DCLK1-GFP was also present in spines ( Fig. 1j ). Measurement of DCLK immunoreactivity and its relative abundance against a soluble volume marker GFP indicated that, although DCLK proteins were present in spines, their enrichment in spines was not high. DCLK proteins were also present in the Triton-treated PSD fraction, but their content was lower than that of PSD-95 ( Fig. 1k ). Because sarkosyl treatment of PSD fraction resulted in a large decrease in DCLK content, interaction of DCLK proteins with the PSD core proteins may not be strong. Interaction between DCLK proteins and PSD scaffolds was further confirmed by immunoprecipitation ( Fig. 1l ). These results indicate the presence of DCLK proteins in the postsynaptic cytoplasm and suggest a possible interaction with PSD proteins. DCLK overexpression enhances dendritic growth The distal-to-proximal concentration gradient of DCLK in dendrites at 7 DIV suggests active roles for DCLK proteins in dendritic growth. To analyse this, we first adopted a gain-of-function strategy and evaluated the effects of DCLK1 (long form) overexpression by transfection of DCLK1-GFP plus lacZ at 8 DIV and subsequent fixation at 14 DIV ( Fig. 2a ). The morphology of dendrites was visualized by anti-β-galactosidase immunostaining and was evaluated by Sholl analysis. Neurons overexpressing DCLK1-GFP showed a significant increase in dendritic complexity ( Fig. 2c ) and the total dendritic length ( Fig. 2d ). 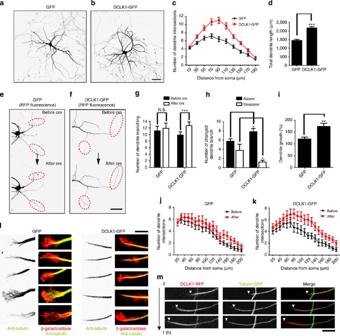Figure 2: Regulation of dendritic growth by DCLKs. (a,b) Dissociated hippocampal neurons expressing GFP or DCLK1-GFP from 8 to 14 DIV. Note the more complex dendritic branching in neurons expressing DCLK1-GFP. (c,d) Sholl analysis and total dendritic lengths of neurons expressing GFP or DCLK1-GFP (number of cells analysed; GFP: 30 and DCLK1-GFP: 30;t-test: ***P<0.001). (e,f) Comparison of dendritic morphology before and after induction of DCLK1-GFP or GFP only, by Cre-dependent excision of loxp-stop-loxp sequences. The images before and 3 days after application of Cre-expressing recombinant adenoviruses were recorded (12 and 15 DIV). Prominent upregulation of dendritic growth was observed only in neurons expressing DCLK1-GFP (red dotted circles). (g) The total number of dendritic branches per neurons was significantly increased in neurons after induction of DCLK1-GFP expression. (number of cells analysed; GFP: 9 and DCLK1-GFP: 13;t-test: ***P<0.001.) (h) Overexpression of DCLK1-GFP suppressed pruning of dendrites and increased the rate of appearance of new dendritic segments (number of cells analysed; GFP: 9 and DCLK1-GFP: 13;t-test: *P<0.05). (i) The total length of dendrites per neurons was significantly increased in neurons overexpressing DCLK1-GFP. (Dendritic growth (%)=sum of dendritic length (after)/sum of dendritic length (before)) (Number of cells analysed; GFP: 9 and DCLK1-GFP: 13;t-test: **P<0.01). (j,k) Sholl analyses of neurons before and after induction of GFP (j) or DCLK1-GFP expression (k) (number of cells analysed; GFP: 9 and DCLK1-GFP: 13). (l) Anti-α-tubulin immunnostaining of growth-cone MTs in neurons transfected with plasmids expressing GFP or DCLK1-GFP. DCLK1-GFP expression induced tightly bundled MTs within growth cones. (m) Time-lapse imaging of both DCLK1-RFP and tubulin-GFP. DCLK1-positive segments show proximal to distal translocation in dendrites. Arrowheads indicate the distal end of the DCLK1-positive segment. All numeric data are given as mean±s.e.m. Bar, 50 μm fora,b,eandf; 5 μm forlandm. Figure 2: Regulation of dendritic growth by DCLKs. ( a , b ) Dissociated hippocampal neurons expressing GFP or DCLK1-GFP from 8 to 14 DIV. Note the more complex dendritic branching in neurons expressing DCLK1-GFP. ( c , d ) Sholl analysis and total dendritic lengths of neurons expressing GFP or DCLK1-GFP (number of cells analysed; GFP: 30 and DCLK1-GFP: 30; t -test: *** P <0.001). ( e , f ) Comparison of dendritic morphology before and after induction of DCLK1-GFP or GFP only, by Cre-dependent excision of loxp-stop-loxp sequences. The images before and 3 days after application of Cre-expressing recombinant adenoviruses were recorded (12 and 15 DIV). Prominent upregulation of dendritic growth was observed only in neurons expressing DCLK1-GFP (red dotted circles). ( g ) The total number of dendritic branches per neurons was significantly increased in neurons after induction of DCLK1-GFP expression. (number of cells analysed; GFP: 9 and DCLK1-GFP: 13; t -test: *** P <0.001.) ( h ) Overexpression of DCLK1-GFP suppressed pruning of dendrites and increased the rate of appearance of new dendritic segments (number of cells analysed; GFP: 9 and DCLK1-GFP: 13; t -test: * P <0.05). ( i ) The total length of dendrites per neurons was significantly increased in neurons overexpressing DCLK1-GFP. (Dendritic growth (%)=sum of dendritic length (after)/sum of dendritic length (before)) (Number of cells analysed; GFP: 9 and DCLK1-GFP: 13; t -test: ** P <0.01). ( j , k ) Sholl analyses of neurons before and after induction of GFP ( j ) or DCLK1-GFP expression ( k ) (number of cells analysed; GFP: 9 and DCLK1-GFP: 13). ( l ) Anti-α-tubulin immunnostaining of growth-cone MTs in neurons transfected with plasmids expressing GFP or DCLK1-GFP. DCLK1-GFP expression induced tightly bundled MTs within growth cones. ( m ) Time-lapse imaging of both DCLK1-RFP and tubulin-GFP. DCLK1-positive segments show proximal to distal translocation in dendrites. Arrowheads indicate the distal end of the DCLK1-positive segment. All numeric data are given as mean±s.e.m. Bar, 50 μm for a , b , e and f ; 5 μm for l and m . Full size image The morphology of dendrites before and after expression of exogenous DCLK1-GFP was compared using the Cre- loxp system. Primary neurons were transfected with an expression plasmid containing a β-actin promoter, intervening loxp-stop-loxp sequences, and the downstream DCLK1-GFP cDNA, together with an red fluorescent protein (RFP)-expression plasmid at 4 DIV. After first acquiring images of RFP-positive dendrites at 12 DIV, we expressed Cre recombinase by using adenoviruses, to initiate expression of DCLK1-GFP. We confirmed induction of DCLK1-GFP 3 days after Cre-adenovirus infection and then again recorded images of the same RFP-filled dendrites ( Fig. 2e ). The basic pattern of dendritic arborization was already established at 12 DIV, and control neurons did not show significant increase in the number of dendritic branching from 12 DIV to 15 DIV ( Fig. 2e ). Induction of DCLK1-GFP expression increased the branch number significantly ( Fig. 2g ), enhanced development of new dendritic branches, as well as suppressed pruning of pre-existing branches ( Fig. 2h ), and increased the total length of newly formed dendrites ( Fig. 2i ). Sholl analysis of dendritic complexity confirmed an increase in dendritic branching by induced expression of DCLK1-GFP ( Fig. 2j ). Preferential interaction of DCLKs and MTs in distal dendritic segments may induce bundling of MTs, and thereby directly drive the extension of the dendrites ( Supplementary Fig. S3 ). To test this possibility, MTs in dendritic growth cones were visualized by anti-tubulin staining. Although growth cones of control neurons frequently contained dispersed MTs, most growth cones of neurons overexpressing DCLK1-GFP showed tightly bundled MTs, sometimes penetrating into growth-cone filopodia ( Fig. 2l ). Time-lapse imaging of neurons expressing DCLK1-RFP together with tubulin-GFP revealed tight coupling between MT bundling and DCLK1 association with MTs within the distal dendritic segment ( Fig. 2m ). The DCLK1-enriched domain showed anterograde movement while maintaining its location at the distal segments of MT bundles. These results suggest recruitment of DCLK1 to newly polymerized MTs within growth cones and subsequent induction of MT bundles, which may support further extension of the dendrites. Time-lapse imaging of DCLK1-GFP together with RFP confirmed correlation between bundling of MTs decorated by DCLK1-GFP and dendritic growth as detected by RFP fluorescence ( Supplementary Fig. S4 ). These results are consistent with the concept that DCLK1-dependent polymerization of MTs directly drives rapid growth of distal dendritic segments. DCLK knockdown suppresses dendritic growth To verify the roles of endogenous DCLK proteins in dendrite morphogenesis, we next performed loss-of-function analysis. We used RNAi and used vector-derived short hairpin RNAs (shRNAs) to suppress expression of DCLK1 and DCLK2 selectively ( Fig. 3a , Supplementary Fig. S5A ). Transfection of DCLK1 and DCLK2 shRNA plasmids did not affect DCX expression ( Supplementary Fig. S5B ). DCLK1 shRNA was designed to suppress DCLK1 isoforms containing a DCX domain [17] . DCLK2 shRNA sequence was also designed to be within a DCX domain and should be effective in suppression of two major splice isoforms. Neurons transfected with shRNA plasmids at 4 DIV showed severe impairment of dendritic growth at 9 DIV ( Fig. 3c ), which was confirmed by Sholl analysis ( Fig. 3d ) and the measurement of total dendritic lengths ( Fig. 3e ). The effect on axon lengths was less severe ( Fig. 3f ). The dendritic phenotype was rescued by expression of RNAi-resistant forms of DCLK1 and DCLK2, indicating specificity of the knockdown ( Fig. 3d ). Rescue of the DCLK1-knockdown phenotype by DCLK2 expression suggests their functional redundancy. Thus, both gain-of-function and loss-of-function analyses supported the hypothesis that DCLK1 is essential for dendritic morphogenesis. 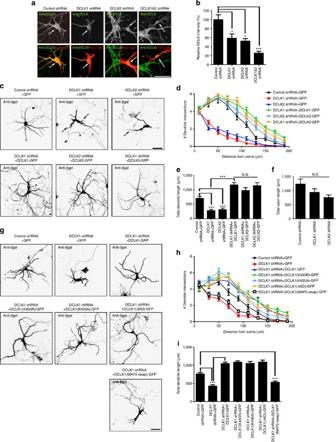Figure 3: Dendritic growth was negatively regulated by DCLK shRNAs. (a,b) Expression of DCLK1 and DCLK2 shRNA plasmids in dissociated hippocampal neurons from 4 to 9 DIV (a). A marked decrease of DCLK immunoreactivity was observed (b) (number of cells analysed; control: 5, DCLK1 shRNA: 6, DCLK2 shRNA: 5, DCLK1 and DCLK2 shRNA: 5; one-way analysis of variance (ANOVA) followed by Tukey–Kramer multiple comparison tests: *P<0.05, ***P<0.001). (c) Neurons transfected with plasmids expressing DCLK1 and DCLK2 shRNAs showed severe impairment of dendritic growth (arrows), which could be rescued by expression of shRNA-resistant constructs for DCLK1 and 2. (d) Sholl analysis of dendritic complexity in neurons transfected with control, DCLK1 shRNA or DCLK2 shRNA plasmids, with or without rescue constructs (number of cells analysed; control: 31, DCLK1 shRNA: 29, DCLK2 shRNA: 30, DCLK1 shRNA plus DCLK1-GFP: 20, DCLK1 shRNA plus DCLK2-GFP: 19 and DCLK2 shRNA plus DCLK2-GFP: 20). (e) Total dendritic lengths of neurons expressing DCLK1 shRNAs or DCLK2 shRNAs, with or without rescue constructs (numbers of cells analysed were the same as ind; one-way ANOVA followed by Tukey–Kramer multiple comparison tests: ***P<0.001). NS, no statistical difference. (f) Total axonal lengths of neurons expressing DCLK1 shRNAs or DCLK2 shRNAs. Total axonal length measured at 5 DIV showed a tendency for reduction without statistical significance (number of cells analysed; control: 30, DCLK1 shRNA: 29 and DCLK2 shRNA: 28). (g) Neurons transfected with DCLK1 shRNA plasmid and expression vectors for various mutants of GFP-tagged DCLK1. Dendritic morphology was visualized by anti-β-galactosidase immunostaining. (h,i) Sholl analyses of dendritic complexity (h) and evaluation of total dendritic length (i) in neurons expressing DCLK1 shRNA plasmid together with expression vectors for various mutants of GFP-tagged DCLK1 (number of cells analysed; control shRNA+GFP: 32, DCLK1 shRNA+GFP: 30, sh+DCLK1-GFP: 27, sh+DCLK1(K435R)-GFP: 27, sh+DCLK1(K435A)-GFP: 28, sh+DCLK1(ΔKD)-GFP: 30 and sh+DCLK1(MAP2 swap)-GFP: 32; one-way ANOVA followed by Tukey–Kramer multiple comparison tests: ***P<0.001). All numeric data are given as mean±s.e.m. Bar, 50 μm fora,candg. Figure 3: Dendritic growth was negatively regulated by DCLK shRNAs. ( a , b ) Expression of DCLK1 and DCLK2 shRNA plasmids in dissociated hippocampal neurons from 4 to 9 DIV ( a ). A marked decrease of DCLK immunoreactivity was observed ( b ) (number of cells analysed; control: 5, DCLK1 shRNA: 6, DCLK2 shRNA: 5, DCLK1 and DCLK2 shRNA: 5; one-way analysis of variance (ANOVA) followed by Tukey–Kramer multiple comparison tests: * P <0.05, *** P <0.001). ( c ) Neurons transfected with plasmids expressing DCLK1 and DCLK2 shRNAs showed severe impairment of dendritic growth (arrows), which could be rescued by expression of shRNA-resistant constructs for DCLK1 and 2. ( d ) Sholl analysis of dendritic complexity in neurons transfected with control, DCLK1 shRNA or DCLK2 shRNA plasmids, with or without rescue constructs (number of cells analysed; control: 31, DCLK1 shRNA: 29, DCLK2 shRNA: 30, DCLK1 shRNA plus DCLK1-GFP: 20, DCLK1 shRNA plus DCLK2-GFP: 19 and DCLK2 shRNA plus DCLK2-GFP: 20). ( e ) Total dendritic lengths of neurons expressing DCLK1 shRNAs or DCLK2 shRNAs, with or without rescue constructs (numbers of cells analysed were the same as in d ; one-way ANOVA followed by Tukey–Kramer multiple comparison tests: *** P <0.001). NS, no statistical difference. ( f ) Total axonal lengths of neurons expressing DCLK1 shRNAs or DCLK2 shRNAs. Total axonal length measured at 5 DIV showed a tendency for reduction without statistical significance (number of cells analysed; control: 30, DCLK1 shRNA: 29 and DCLK2 shRNA: 28). ( g ) Neurons transfected with DCLK1 shRNA plasmid and expression vectors for various mutants of GFP-tagged DCLK1. Dendritic morphology was visualized by anti-β-galactosidase immunostaining. ( h , i ) Sholl analyses of dendritic complexity ( h ) and evaluation of total dendritic length ( i ) in neurons expressing DCLK1 shRNA plasmid together with expression vectors for various mutants of GFP-tagged DCLK1 (number of cells analysed; control shRNA+GFP: 32, DCLK1 shRNA+GFP: 30, sh+DCLK1-GFP: 27, sh+DCLK1(K435R)-GFP: 27, sh+DCLK1(K435A)-GFP: 28, sh+DCLK1(ΔKD)-GFP: 30 and sh+DCLK1(MAP2 swap)-GFP: 32; one-way ANOVA followed by Tukey–Kramer multiple comparison tests: *** P <0.001). All numeric data are given as mean±s.e.m. Bar, 50 μm for a , c and g . Full size image To clarify the involvement of DCLK1 kinase activity in the enhancement of dendrite growth, neurons were transfected with either an RNAi-resistant kinase-dead mutant of DCLK1 (DCLK1 (K435A)-GFP and DCLK1(K435R)-GFP) or an RNAi-resistant DCLK1 without a kinase domain (DCLK1(ΔKD)-GFP). These mutants could rescue the dendritic phenotype of DCLK1 knockdown ( Fig. 3g–i ). Next, we replaced the MT-binding domain of RNAi-resistant DCLK1 with that of MAP2, a major dendritic MAP, and tested the ability of this chimeric molecule (DCLK1(MAP2 swap)-GFP) in promoting dendritic growth. Although DCLK1(MAP2 swap)-GFP could interact with MTs and induce MT bundles in non-neuronal cells ( Supplementary Fig. S3 ), expression of DCLK1(MAP2 swap)-GFP could not rescue the phenotype of DCLK1 knockdown in neurons ( Fig. 3g–i ), indicating the essential role of the DCLK1 MT-binding domain in the promotion of dendritic growth. DCLK regulates postsynaptic structural growth The presence of DCLKs in biochemically purified PSD fraction suggests their postsynaptic function. Expression of DCLK1-GFP by recombinant adenoviruses for 2 days resulted in significant reduction of PSD-95 immunoreactivity ( Fig. 4a ). DCLK1 overexpression did not induce strong reduction in PSD-95 puncta density, but was effective in reducing the density of VGLUT1-positive presynaptic puncta ( Supplementary Fig. S6A–D ). The reduction of the PSD-95 signal was not due to an overall reduction of the PSD-95 protein level ( Supplementary Fig. S7 ). Furthermore, the density of total dendritic spines was reduced in neurons expressing DCLK1-GFP ( Fig. 4c ), together with the fraction of mushroom spines ( Fig. 4e ). These results indicate that excitatory synaptic development is negatively regulated by DCLK1 (long form). 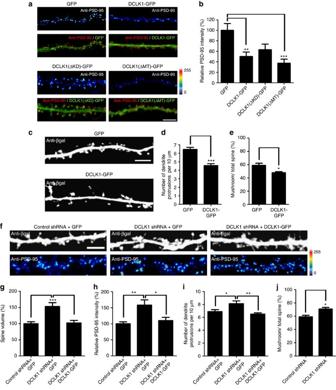Figure 4: Regulation of postsynaptic functions by DCLK1. (a,b) Fluorescence images of dendrites expressing GFP, DCLK1-GFP, GFP-tagged DCX domain of DCLK1 (DCLK1(ΔKD)-GFP) or GFP-tagged kinase domain of DCLK1 (DCLK1(ΔMT)-GFP) (a). Neurons expressed the various forms of DCLKs from 18 to 20 DIV. Prominent reduction of PSD-95 immunoreactivity was observed in neurons overexpressing DCLK1-GFP or DCLK1(ΔMT)-GFP (b) (number of cells analysed; GFP: 19, DCLK1-GFP: 20, DCLK1(ΔKD)-GFP: 20 and DCLK1(ΔMT)-GFP: 20; one-way analysis of variance (ANOVA) followed by Tukey–Kramer multiple comparison tests: **P<0.01, ***P<0.001). (c–e) Anti-β-galactosidase staining of neurons expressing either GFP only or DCLK1-GFP (c). Density of dendritic protrusions was significantly reduced in DCLK1-GFP-expressing neurons (d) and the fraction of mushroom-type spines was also reduced (e) (number of cells analysed; GFP: 24, DCLK1-GFP: 26;t-test: *P<0.05, ***P<0.001). (f) Anti-β-galactosidase staining and anti-PSD-95 staining of neurons transfected with control shRNA plus GFP-expression plasmids, DCLK1 shRNA plus GFP-expression plasmid or DCLK1 shRNA plus shRNA-resistant DCLK1-GFP-expression plasmids. LacZ expression plasmids were included in all transfection experiments for the purpose of volume label. (g–j) Effects of DCLK1 knockdown on spines and PSDs. Neurons expressing DCLK1 shRNAs showed significant increase of spine volume (g) and the total intensity of PSD-95 clusters (h). These neurons also showed a slight, but significant, increase of dendritic protrusion density (i). Classification of spine types revealed increase in the fraction of mushroom-type spines (j). These effects of DCLK1 knockdown were rescued by expression of shRNA-resistant DCLK1-GFP (number of cells analysed; control: 20, DCLK1 shRNA: 18 and DCLK1 shRNA plus shRNA-resistant DCLK1: 20; one-way ANOVA followed by Tukey–Kramer multiple comparison tests ort-test: *P<0.05, **P<0.01, ***P<0.001) All numeric data are given as mean±s.e.m. Bar, 5 μm fora; 10 μm forcandf. Figure 4: Regulation of postsynaptic functions by DCLK1. ( a , b ) Fluorescence images of dendrites expressing GFP, DCLK1-GFP, GFP-tagged DCX domain of DCLK1 (DCLK1(ΔKD)-GFP) or GFP-tagged kinase domain of DCLK1 (DCLK1(ΔMT)-GFP) ( a ). Neurons expressed the various forms of DCLKs from 18 to 20 DIV. Prominent reduction of PSD-95 immunoreactivity was observed in neurons overexpressing DCLK1-GFP or DCLK1(ΔMT)-GFP ( b ) (number of cells analysed; GFP: 19, DCLK1-GFP: 20, DCLK1(ΔKD)-GFP: 20 and DCLK1(ΔMT)-GFP: 20; one-way analysis of variance (ANOVA) followed by Tukey–Kramer multiple comparison tests: ** P <0.01, *** P <0.001). ( c – e ) Anti-β-galactosidase staining of neurons expressing either GFP only or DCLK1-GFP ( c ). Density of dendritic protrusions was significantly reduced in DCLK1-GFP-expressing neurons ( d ) and the fraction of mushroom-type spines was also reduced ( e ) (number of cells analysed; GFP: 24, DCLK1-GFP: 26; t -test: * P <0.05, *** P <0.001). ( f ) Anti-β-galactosidase staining and anti-PSD-95 staining of neurons transfected with control shRNA plus GFP-expression plasmids, DCLK1 shRNA plus GFP-expression plasmid or DCLK1 shRNA plus shRNA-resistant DCLK1-GFP-expression plasmids. LacZ expression plasmids were included in all transfection experiments for the purpose of volume label. ( g – j ) Effects of DCLK1 knockdown on spines and PSDs. Neurons expressing DCLK1 shRNAs showed significant increase of spine volume ( g ) and the total intensity of PSD-95 clusters ( h ). These neurons also showed a slight, but significant, increase of dendritic protrusion density ( i ). Classification of spine types revealed increase in the fraction of mushroom-type spines ( j ). These effects of DCLK1 knockdown were rescued by expression of shRNA-resistant DCLK1-GFP (number of cells analysed; control: 20, DCLK1 shRNA: 18 and DCLK1 shRNA plus shRNA-resistant DCLK1: 20; one-way ANOVA followed by Tukey–Kramer multiple comparison tests or t -test: * P <0.05, ** P <0.01, *** P <0.001) All numeric data are given as mean±s.e.m. Bar, 5 μm for a ; 10 μm for c and f . Full size image To determine whether endogenous DCLK1 also negatively regulates spine structure and PSD-95 accumulation, neurons were transfected with DCLK1 shRNA plasmids at 9 DIV, and multiple parameters of synapse maturation were measured at 14 DIV (spine volume, PSD-95 immunoreactivity, spine density and the fraction of mushroom spines were shown in Fig. 4f–j ; PSD-95 and VGLUT1 puncta densities were shown in Supplementary Fig. S6E–H ). Although the increases in spine density and the fraction of mushroom spines were moderate ( Fig. 4i ), spine volume, PSD-95 immunoreactivity and PSD-95 puncta density increased significantly ( Fig. 4g , Supplementary Fig. S6F ). The phenotypes of DCLK1 knockdown were rescued by expression of an RNAi-resistant form of DCLK1, indicating specificity of the knockdown ( Fig. 4f–i ). Transfection of DCLK1 shRNA at 9 DIV did not result in obvious impairment of dendritic growth, indicating that reduction of the DCLK1 level does not induce shrinkage of pre-existing dendrites. Thus, both overexpression and knockdown experiments suggested negative regulation of the postsynaptic structural growth by DCLK1. Two distinct pathways in synapse regulation by DCLKs We next evaluated the effect of expressing the DCX domain or the kinase domain, fused to GFP, on the content of PSD-95 in dendrites. Overexpression of the kinase domain reduced the content of PSD-95 to 38% of that in the control neurons ( Fig. 4a ). Another scaffolding protein, Homer, showed a similar tendency in neurons transfected with DCLK1 variants ( Supplementary Fig. S8 ). These results are consistent with the concept that, in addition to the role of regulating MTs via the DCX domain, DCLK proteins have a role in the negative regulation of the postsynaptic protein content through the kinase domain. The neurons expressing the DCX domain showed a tendency for decreased PSD-95 expression ( Fig.4a ), suggesting an additional role of the DCX domain in postsynaptic function. To test this possibility, we expressed wild-type or truncated forms of DCLK1 by using recombinant adenoviruses from 15 DIV to 17 DIV and detailed morphology of spines were evaluated by DiI staining ( Fig. 5a ). Overexpression of the GFP-tagged full-length DCLK1 enhanced generation of long and thin dendritic protrusions. This effect was maintained when the GFP-tagged DCX domain was expressed, but abolished in neurons expressing the GFP-tagged kinase domain ( Fig. 5a–c ). These results indicate a specific role for the DCX domain in formation and morphological maturation of spines. 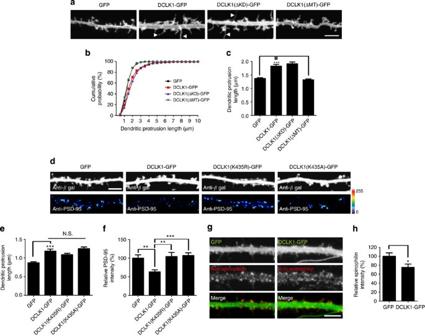Figure 5: Roles of DCLK1 domains on postsynaptic functions. (a) Morphology of dendrites labelled by DiI. Effects of overexpressing either GFP alone, wild-type DCLK1-GFP, the GFP-tagged DCX domain of DCLK1 (DCLK1(ΔKD)-GFP) or the GFP-tagged kinase domain of DCLK1 (DCLK1(ΔMT)-GFP) were evaluated. (b) Cumulative curves of spine/filopodia length in neurons expressing either GFP only, full-length DCLK1-GFP, DCLK1(ΔKD)-GFP or DCLK1(ΔMT)-GFP (GFP:n=6 cells, 300 spines; DCLK1-GFP:n=7cells, 350 spines; DCLK1(ΔKD)-GFP:n=6 cells, 300 spines; and DCLK1(ΔMT)-GFP:n=6 cells, 300 spines). (c) Length of dendritic protrusions in neurons expressing GFP only, full-length DCLK1-GFP, DCLK1(ΔKD)-GFP or DCLK1(ΔMT)-GFP (number of cells and spines analysed were the same as inb; one-way analysis of variance (ANOVA) followed by Tukey–Kramer multiple comparison tests: ***P<0.001). (d) Morphology of dendritic protrusions and PSD-95 immunoreactivity in neurons expressing GFP only, DCLK1-GFP and the GFP-tagged DCLK1 with kinase-dead point mutations (DCLK1 (K435R)-GFP and DCLK1 (K435A)-GFP). (e,f) Length of dendritic protrusions (e) and relative intensity of PSD-95 puncta (f) in neurons expressing GFP only, DCLK1-GFP, DCLK1 (K435R)-GFP and DCLK1 (K435A)-GFP (GFP:n=30 cells, 1033 spines; DCLK1-GFP:n=29 cells, 985 spines; DCLK1 (K435R)-GFP:n=14 cells, 510 spines; and DCLK1 (K435A)-GFP:n=20 cells, 657 spines; one-way ANOVA followed by Tukey–Kramer multiple comparison tests: **P<0.01, ***P<0.001). (g) Reduction of spinophilin content in dendrites by overexpression of DCLK1-GFP. (h) Quantification of spinophilin immunoreactivity in spines revealed suppression of spinophilin expression in neurons expressing DCLK1-GFP (GFP:n=19 and DCLK1-GFP:n=18;t-test: *P<0.05). All numeric data are given as mean±s.e.m. Bar, 5 μm fora,dandg. Figure 5: Roles of DCLK1 domains on postsynaptic functions. ( a ) Morphology of dendrites labelled by DiI. Effects of overexpressing either GFP alone, wild-type DCLK1-GFP, the GFP-tagged DCX domain of DCLK1 (DCLK1(ΔKD)-GFP) or the GFP-tagged kinase domain of DCLK1 (DCLK1(ΔMT)-GFP) were evaluated. ( b ) Cumulative curves of spine/filopodia length in neurons expressing either GFP only, full-length DCLK1-GFP, DCLK1(ΔKD)-GFP or DCLK1(ΔMT)-GFP (GFP: n =6 cells, 300 spines; DCLK1-GFP: n =7cells, 350 spines; DCLK1(ΔKD)-GFP: n =6 cells, 300 spines; and DCLK1(ΔMT)-GFP: n =6 cells, 300 spines). ( c ) Length of dendritic protrusions in neurons expressing GFP only, full-length DCLK1-GFP, DCLK1(ΔKD)-GFP or DCLK1(ΔMT)-GFP (number of cells and spines analysed were the same as in b ; one-way analysis of variance (ANOVA) followed by Tukey–Kramer multiple comparison tests: *** P <0.001). ( d ) Morphology of dendritic protrusions and PSD-95 immunoreactivity in neurons expressing GFP only, DCLK1-GFP and the GFP-tagged DCLK1 with kinase-dead point mutations (DCLK1 (K435R)-GFP and DCLK1 (K435A)-GFP). ( e , f ) Length of dendritic protrusions ( e ) and relative intensity of PSD-95 puncta ( f ) in neurons expressing GFP only, DCLK1-GFP, DCLK1 (K435R)-GFP and DCLK1 (K435A)-GFP (GFP: n =30 cells, 1033 spines; DCLK1-GFP: n =29 cells, 985 spines; DCLK1 (K435R)-GFP: n =14 cells, 510 spines; and DCLK1 (K435A)-GFP: n =20 cells, 657 spines; one-way ANOVA followed by Tukey–Kramer multiple comparison tests: ** P <0.01, *** P <0.001). ( g ) Reduction of spinophilin content in dendrites by overexpression of DCLK1-GFP. ( h ) Quantification of spinophilin immunoreactivity in spines revealed suppression of spinophilin expression in neurons expressing DCLK1-GFP (GFP: n =19 and DCLK1-GFP: n =18; t -test: * P <0.05). All numeric data are given as mean±s.e.m. Bar, 5 μm for a , d and g . Full size image To further confirm the role of kinase activity in synapse regulation, neurons were transfected with kinase-dead DCLK1 mutants (K435R or K435A amino-acid substitutions) together with lacZ and stained with anti-PSD-95 and anti-β-galactosidase antibodies ( Fig. 5d ). Kinase-dead DCLK1 mutants enhanced generation of long and thin dendritic protrusions ( Fig. 5e ), but did not suppress the synaptic content of PSD-95 ( Fig. 5f ), suggesting a selective role for DCLK1 kinase activity in accumulation of PSD-95. The selective role of DCLK1 kinase activity in PSD-95 accumulation was further confirmed by overexpression of DCLK1 kinase domain with kinase-dead mutations ( Supplementary Fig. 9 ). Previous studies reported interaction of DCLK1 with spinophilin, an actin-binding protein known to regulate spine morphology. We performed spinophilin immunocytochemistry of neurons overexpressing DCLK1-GFP ( Fig. 5g ) and found reduction of spinophilin content ( Fig. 5h ). Because previous studies reported induction of excess filopodia in spinophilin-knockout mice [18] , the increase in long and thin dendritic protrusions observed in DCLK1-GFP-overexpressing neurons could be explained by reduction of postsynaptic spinophilin content. DCLK1 regulates functions of glutamatergic synapses The exogenous overexpression of DCLK1-GFP caused a reduction in the synaptic content of PSD-95 and morphological alteration of spines. We next evaluated the effect of DCLK1 overexpression on synaptic transmission by recording miniature excitatory postsynaptic currents (mEPSCs) from DCLK1-GFP-overexpressing neurons ( Fig. 6a ). The amplitude of mEPSCs was decreased in neurons expressing DCLK1-GFP ( Fig. 6b ) and the inter-event interval was increased ( Fig. 6c ). 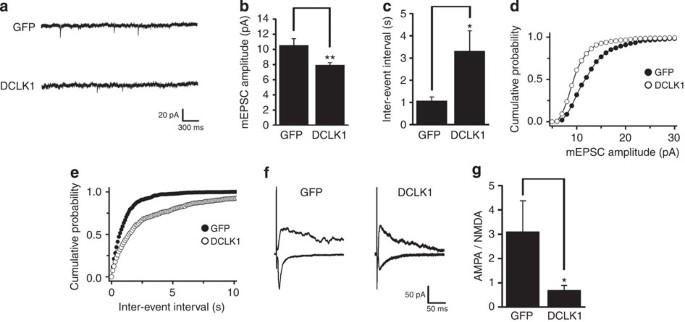Figure 6: Regulation of AMPA receptor-mediated current by DCLK1. (a–e) mEPSC traces (a). Scale bar, 20 pA, 300 ms. The average and cumulative distribution of mEPSC amplitudes (b,d) and inter-event intervals (c,e) recorded from dissociated hippocampal neurons. Overexpression of DCLK1-GFP by infection of recombinant adenoviruses induced a decrease in mEPSC amplitudes and increase in inter-event intervals. (GFP:n=6 cells and DCLK1-GFP:n=8 cells; one-way analysis of variance (ANOVA): *P<0.05, **P<0.01.) (f) Traces of evoked EPSCs from neurons expressing either GFP only or DCLK1-GFP by using recombinant adenoviruses. Scale bar, 50 pA, 50 ms. (g) Mean and s.e.m of the AMPA/NMDA EPSC ratio in neurons overexpressing GFP alone or DCLK1-GFP. The graph shows significant suppression of the AMPA/NMDA EPSC ratio by DCLK1-GFP overexpression (GFP: n=8 cells and DCLK1-GFP:n=11 cells; one-way ANOVA: *P<0.05). All numeric data are given as mean±s.e.m. Figure 6: Regulation of AMPA receptor-mediated current by DCLK1. ( a – e ) mEPSC traces ( a ). Scale bar, 20 pA, 300 ms. The average and cumulative distribution of mEPSC amplitudes ( b , d ) and inter-event intervals ( c , e ) recorded from dissociated hippocampal neurons. Overexpression of DCLK1-GFP by infection of recombinant adenoviruses induced a decrease in mEPSC amplitudes and increase in inter-event intervals. (GFP: n =6 cells and DCLK1-GFP: n =8 cells; one-way analysis of variance (ANOVA): * P <0.05, ** P <0.01.) ( f ) Traces of evoked EPSCs from neurons expressing either GFP only or DCLK1-GFP by using recombinant adenoviruses. Scale bar, 50 pA, 50 ms. ( g ) Mean and s.e.m of the AMPA/NMDA EPSC ratio in neurons overexpressing GFP alone or DCLK1-GFP. The graph shows significant suppression of the AMPA/NMDA EPSC ratio by DCLK1-GFP overexpression (GFP: n=8 cells and DCLK1-GFP: n =11 cells; one-way ANOVA: * P <0.05). All numeric data are given as mean±s.e.m. Full size image The increase in the mEPSC inter-event interval may indicate either a reduced number of synapses, an increased proportion of synapses without an AMPA (a-amino-3-hydroxy-5-methyl-4-isoxazole propionic acid) receptor response (silent synapses) or changes in the presynaptic release probability. Because DCLK is enriched in the postsynaptic compartment, the observed changes in mEPSC amplitude may reflect alterations in the synaptic AMPA receptor content. If this is the case, the ratio of the AMPA receptor-mediated synaptic currents to the NMDA ( N -methyl- D -aspartate) receptor-mediated component should be modulated. To test this, we recorded evoked synaptic responses at both −70 mV and +40 mV and estimated the AMPA/NMDA ratio ( Fig. 6f ). We found that the AMPA/NMDA ratio was reduced to approximately 25% of that of the control neurons ( Fig. 6g ). We further confirmed the reduced synaptic content of AMPA receptors by immunocytochemistry ( Supplementary Fig. S10 ). These results are consistent with the concept that DCLKs regulate both the content of PSD scaffolds and spine morphology, leading to the functional suppression of glutamatergic synaptic transmission. DCLKs regulate dendritic growth and spine morphology in vivo Previous studies of DCLK1 −/− mice revealed intact cortical lamination and migration of the pyramidal neuron precursors [19] , but defects in the formation of axonal tracts [17] . Because the morphology of the dendritic spines in DCLK1 −/− mice had not yet been evaluated, we first performed Golgi staining in the hippocampal CA1 region of DCLK1 +/+ and DCLK1 −/− mice and classified spines into mushroom or thin spines ( Fig. 7a ) [20] . In DCLK1 −/− mice, the fraction of mushroom spines was significantly increased ( Fig. 7b ), suggesting DCLK1-dependent control of spine shape in vivo . 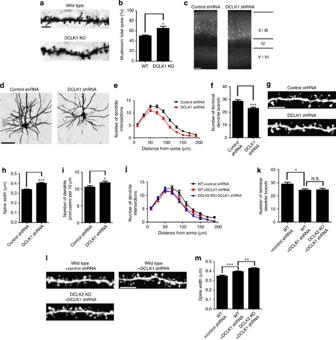Figure 7:In vivophenotypes of DCLK knockdown and knockout. (a,b) Golgi staining of the hippocampal CA1 area prepared from wild-type orDCLK1−/−mice (a) revealed an increase of mushroom-type spines in the latter (b) (WT:n=3 and DCLK1-KO:n=3 (littermates);t-test: *P<0.05) (c) The indistinguishable migratory properties of neuronal precursors in the somatosensory cortex with or without DCLK1 shRNA. (d–f) Cortical pyramidal neuron dendritesin vivoafterin uteroelectroporation of DCLK1 shRNAs (d) showed reduction of dendritic complexity by Sholl analyses (e) and a smaller number of terminal dendritic branches (f) (control:n=45 cells and DCLK1 shRNA:n=45 cells;t-test: ***P<0.001). (g–i) GFP fluorescence of dendritic protrusions in pyramidal neurons afterin uteroelectroporation of DCLK1 shRNAs (g) revealed an increase in spine width (h) and spine density (i) (control:n=18 cells, 624 spines and DCLK1 shRNA:n=17 cells, 501 spines;t-test: *P<0.05, ***P<0.001). (j,k) Manipulation of DCLK1 expression on theDCLK2−/−genetic background did not enhance impairment of dendritic growth. The complexity of dendrites (j) and the number of total terminal dendritic branches (k) were analysed in cortical pyramidal neurons expressing control or DCLK1 shRNAs on wild-type orDCLK2−/−background (WT+control shRNA:n=22 cells; WT+DCLK1 shRNA:n=17 cells; andDCLK2-KO+DCLK1 shRNA:n=21 cells; one-way analysis of variance (ANOVA) followed by Tukey–Kramer multiple comparison tests: *P<0.05). NS, no statistical difference. (l,m) Expression of DCLK1 shRNAs on aDCLK2−/−genetic background further enhanced the increase in spine widths (WT+control shRNA:n=22 cells, 768 spines; WT+DCLK1 shRNA:n=17 cells, 622 spines;DCLK2-KO+DCLK1 shRNA:n=20 cells, 802 spines; one-way ANOVA followed by Tukey–Kramer multiple comparison tests: **P<0.01,***P<0.001). All numeric data are given as mean±s.e.m. Bar, 5 μm fora,gandl; 100 μm forc; and 50 μm ford. Figure 7: In vivo phenotypes of DCLK knockdown and knockout. ( a , b ) Golgi staining of the hippocampal CA1 area prepared from wild-type or DCLK1 −/− mice ( a ) revealed an increase of mushroom-type spines in the latter ( b ) (WT: n =3 and DCLK1-KO: n =3 (littermates); t -test: * P <0.05) ( c ) The indistinguishable migratory properties of neuronal precursors in the somatosensory cortex with or without DCLK1 shRNA. ( d – f ) Cortical pyramidal neuron dendrites in vivo after in utero electroporation of DCLK1 shRNAs ( d ) showed reduction of dendritic complexity by Sholl analyses ( e ) and a smaller number of terminal dendritic branches ( f ) (control: n =45 cells and DCLK1 shRNA: n =45 cells; t -test: *** P <0.001). ( g – i ) GFP fluorescence of dendritic protrusions in pyramidal neurons after in utero electroporation of DCLK1 shRNAs ( g ) revealed an increase in spine width ( h ) and spine density ( i ) (control: n =18 cells, 624 spines and DCLK1 shRNA: n =17 cells, 501 spines; t -test: * P <0.05, *** P <0.001). ( j , k ) Manipulation of DCLK1 expression on the DCLK2 −/− genetic background did not enhance impairment of dendritic growth. The complexity of dendrites ( j ) and the number of total terminal dendritic branches ( k ) were analysed in cortical pyramidal neurons expressing control or DCLK1 shRNAs on wild-type or DCLK2 −/− background (WT+control shRNA: n =22 cells; WT+DCLK1 shRNA: n =17 cells; and DCLK2 -KO+DCLK1 shRNA: n =21 cells; one-way analysis of variance (ANOVA) followed by Tukey–Kramer multiple comparison tests: * P <0.05). NS, no statistical difference. ( l , m ) Expression of DCLK1 shRNAs on a DCLK2 −/− genetic background further enhanced the increase in spine widths (WT+control shRNA: n =22 cells, 768 spines; WT+DCLK1 shRNA: n =17 cells, 622 spines; DCLK2 -KO+DCLK1 shRNA: n =20 cells, 802 spines; one-way ANOVA followed by Tukey–Kramer multiple comparison tests: ** P <0.01,*** P <0.001). All numeric data are given as mean±s.e.m. Bar, 5 μm for a , g and l ; 100 μm for c ; and 50 μm for d . Full size image The spine phenotype in DCLK1 −/− mice may not be associated with postsynaptic DCLK1 functions, but may be derived from defects in the hippocampal commissure tracts. To clarify the cell-autonomous effects of DCLK1 suppression in vivo , we knocked down DCLK1 in neocortical pyramidal neurons by in utero electroporation of DCLK1 shRNA plasmids. Although defects in radial migration of neocortical pyramidal neuron precursors by RNAi-mediated knockdown of DCLK1 at embryonic day 13.5 have been reported [17] , neural precursors transfected with DCLK1 shRNA plasmids at E15.5 settled within layer II-III of the neocortex in a manner indistinguishable from that of the control neurons ( Fig. 7c ). To visualize the dendritic arborization of single pyramidal neurons, we utilized the technique of promoter-assisted sparse-neuron multiple-gene labelling using in utero electroporation (PASME; see Methods for detail) [21] . This method enabled us to label layer II-III pyramidal neurons sparsely at 3 weeks after birth and trace the complex dendritic branches reliably ( Fig. 7d ). Sholl analysis and counting the number of terminal dendritic branches indicated reduced dendritic complexity in neurons expressing DCLK1 shRNA ( Fig. 7e ). Spines on the apical dendritic branches were wider than those on control dendrites ( Fig. 7g ), but the density of dendritic spines was only moderately increased ( Fig. 7i ). By applying PASME technique to the hippocampal neurons, we could confirm dual effects of DCLK1 shRNA on dendritic arborization and spine morphology ( Supplementary Fig. S11D–H ). Thus, the in vivo knockdown approach confirmed the role of DCLK1 in both inhibition of spine growth and enhancement of dendritic complexity. We further confirmed that neocortical pyramidal neurons in DCLK1 −/− mice show suppressed growth of dendrites by applying PASME to DCLK1 −/− mice and expressed GFP in a small subset of pyramidal neurons ( Supplementary Fig. S11A–C ). We next tested whether further deletion of DCLK2 may have an additive effect on enhancement of dendritic complexity and inhibition of spine growth. For this purpose, we repeated in utero electroporation of DCLK1 shRNA plasmids on the genetic background of DCLK2 −/− . It had been shown previously that DCLK2 single-knockout mice demonstrated no obvious defects in brain architecture [22] . When DCLK1 was downregulated by shRNAs, absence of DCLK2 did not induce further reduction of dendritic complexity ( Fig. 7j ). However, the effect on spine morphology was further enhanced in the absence of DCLK2 ( Fig. 7l ). These results suggest that the dosage of multiple DCLK genes contributes to spine volume regulation. Our biochemical and immunocytochemical analyses showed persistent expression of DCLK proteins in postmitotic neurons. DCLK1 (long form) is expressed in both embryonic and adult brains [17] , whereas the expression of DCLK1 (short form) is increased in adult brain [11] , [23] . The third variant (DCL) is composed of the DCX domain plus the Ser-Pro-rich linker; its expression is reported to be downregulated postnatally [17] , but a recent report indicated abundance of this isoform in a specific subset of neuronal cells in the adult brain [24] . The balance between DCLK1 (short form) and DCL expression may precisely regulate postsynaptic functions, because these variants have distinct roles in PSD accumulation and spine morphogenesis. Further analysis of expression profiles in various neuron subtypes may clarify the DCLK-dependent mechanisms of postsynaptic maturation. Live imaging revealed tight temporal coupling of dendrite growth, decoration of MTs by DCLK1 and bundling of MTs in the distal dendritic segments. Recently, similar roles of DCLK1 in growth-cone MTs of sympathetic neurons were proposed [25] . MT-binding regions of DCX and DCLK1 are composed of two tandem homologous domains, with differential affinity for assembled MTs and tubulin dimers [3] , [26] , [27] . Our study showed that replacement of the DCLK1 MT-binding domain with that of MAP2, which lacked the ability to interact with tubulin dimers [28] , eliminated the capacity for dendritic growth promotion. Thus, the ability of DCLK1 to interact with tubulin dimers may have an essential role in the enhancement of dendritic growth, probably by initiating assembly of new MTs. In addition to the impairment of dendritic growth, DCLK1- and DCX/DCLK1-deficient neurons showed specific defects in axonal projections, such as the absence of the corpus callosum [17] , [19] . In our in vitro experiments, knockdown of DCLK1 and DCLK2 resulted in the reduction of axonal length, but without statistical significance. The possible roles of DCL in the radial process stability of neuronal precursors have been reported [29] , and DCLK proteins may have a critical role in formation of neuronal processes at multiple stages of development. Recent studies suggested essential roles of DCX and DCLK1 in the function of kinesin superfamily protein Kif1a [30] and also transport of glucocorticoid receptors [31] , suggesting diverse roles of DCX and DCLK. We provided evidence of the role of DCLK1 kinase activity in the regulation of postsynaptic functions. Introduction of a single amino-acid substitution into the kinase domain eliminated the ability of DCLK1 to reduce PSD-95 content. To further clarify the underlying mechanism, identification of kinase substrates is essential. However, only a few candidate substrates of DCLK1 have been identified to date [32] , [33] , and future proteomic analysis of phosphoprotein profile in DCLK-mutant mice should be important. Expression of the truncated mutant of the DCX domain increased thin spines, suggesting an additional role of the two DCX repeats in regulation of postsynaptic functions. Interestingly, overexpression of DCLK1 reduces the level of spinophilin, a protein that is known to bind F-actin and regulate spine morphology [34] , [35] . Excess DCLK1 bound to dendritic MTs may trap spinophilin and reduce spinophilin content in spines. Because an increase in filopodia-like structures was observed in dendrites of spinophilin −/− neurons [18] , DCLK1-dependent reduction of spinophilin content may affect spine morphology. Overexpression of DCLK1 results in a reduction of functional AMPA receptors. This postsynaptic effect can be explained by either reduction of synaptic content of PSD-95 (refs 36 , 37 , 38 ) or reduction in spine head volume, which was reported to be coupled to AMPA receptor content [39] , [40] . It is likely that DCLK1 regulates postsynaptic functions through multiple pathways including both kinase-mediated signalling and cytoskeletal reorganization. Two functions of DCLKs, MT binding and kinase activity, may be regulated by independent upstream regulators. Cdk5-mediated phosphorylation and protein phosphatase 1-mediated dephosphorylation of DCX at Ser297 are important in regulation of its affinity to MTs [41] , [42] . Because the amino-acid sequences of DCLK1 around Ser298 show high homology with DCX, MT-binding affinity of DCLK1 may also be regulated by Cdk5 and protein phosphatase 1. Kinase activity of DCLK1 is not directly regulated by Ca 2+ -bound CaM (ref. 43 ). DCLK1 kinase activity is upregulated by introducing a phosphorylation-mimic mutation to Thr239, a residue within the activation loop site. Because phosphorylation of Thr177 in CaMKI, which is equivalent to Thr239 of DCLK1, by CaMK kinase enhances CaMKI activity, it has been speculated that DCLK1 kinase activity can be regulated by upstream kinases similar to CaMK kinase [43] . Regulation of dual functions of DCLKs by upstream kinases should be critical in activity-dependent regulation of DCLK-mediated remodelling of dendrites and postsynaptic molecular assembly. In this study, we provided evidence for multiple DCLK functions in dendritic development. DCLK proteins are localized in distal dendrites and enhance their growth. Simultaneously, DCLK proteins enter the spine cytoplasm and suppress PSD-95 accumulation, spine maturation and surface expression of AMPA receptors. This repression of synapse maturation is likely to be important for keeping distal dendrites devoid of mature synapses and enhancing their structural remodelling. Generation of anti-DCLK antibody Residues 54–138 of the amino-acid sequence of mouse DCLK1 (Gene ID 13175) was selected as antigen; this was expressed in Escherichia coli strain BL21 as a recombinant protein and utilized as an antigen for generating rabbit polyclonal antibodies. This antigen did not exist in DCLK3 (refs 6 , 7 ) [6] , [7] , another DCLK that, unlike DCLK1 and DCLK2, is not highly expressed in brain. This antibody also did not react with DCX protein ( Supplementary Fig. S1 ). This antibody was useful in specific detection of DCLK proteins in fixed preparations of both cultured primary neurons and brain sections. Commercially available antibodies that we tested were not as sensitive as this antibody. Other antibodies See Supplementary Methods . Construction of expression plasmids and generation of recombinant adenoviruses The cDNA of mouse wild-type DCLK1 sequence was amplified by PCR and inserted into pEGFP-N1 (Clontech) to generate DCLK1-GFP. DCLK1-mutant constructs were summarized in Supplementary Table S1 . DNA segments corresponding to kinase domain (amino acids 314–757 of DCLK1) or DCX domain (amino acids 1–350 of DCLK1) were also inserted into either pEGFP-N1 or pEGFP-C1 to generate DCLK1(ΔMT)-GFP or DCLK1(ΔKD)-GFP. DCLK1(MAP2 swap)-GFP was generated by replacing the MT-binding domain of DCLK1 (amino acids 1–270) with the MT-binding domain of MAP2C (amino acids 224–499) [44] . DCLK1(K435R)-GFP, DCLK1(K435A)-GFP, DCLK1(ΔMT K435R)-GFP and DCLK1(ΔMT K435A)-GFP were generated by introducing a mutation using the QuickChange Site-Directed Mutagenesis Kit (Stratagene) into full-length DCLK1 or DCLK1(ΔMT), respectively. The cDNA of tubulin N-terminally tagged with GFP (tubulin-GFP) was excised from the pAcGFP1-tubulin vector (Clontech) and inserted into the expression vector under the control of the β-actin promoter. RFP and lacZ reporter plasmids were generated by replacing the GFP-coding region of the pAct-GFP plasmid [45] with the coding region of either lacZ gene (pCMVβ vector; Clontech), DsRed2 (Clontech) or mRFP [46] . The plasmid for expression of DCLK1 with intervening loxp-stop-loxp sequences used in transfection experiments of cultured neurons was generated from the pAct-loxP STOP-GFP plasmid [47] by replacing the GFP sequence with that for DCLK1-GFP. Adenoviruses for the expression of DCLK1-GFP, truncated forms of DCLK1 tagged with GFP and Cre recombinase were constructed and purified as described previously [45] , [48] . RNAi The RNAi-targeting sequence for DCLK1 (5′-GGTTCGATTCTACAGAAAT-3′) was as previously reported [17] . The targeting sequence for DCLK2 (5′-GCAGGTTACTTGTCTGCAAGA-3′) was designed ab initio and its effect was confirmed by co-transfection with DCLK2-GFP. These oligonucleotides were ligated into the shRNA expression vector (pSilencer 2.0-U6; Invitrogen) and transfected into cells using the Effectene transfection reagent (Qiagen). Stealth RNAi Negative Control Duplexes (Invitrogen) were used as control shRNAs. The sequence for a resistant form of DCLK1 was designed by introducing three-point mutations into the original sequences (5′-GGTCCGATTTTACAGGAAT-3′). Western blotting See Supplementary Methods . Biochemical purification of PSDs See Supplementary Methods . Hippocampal neuronal culture and DiI labelling Cell suspensions were prepared from E16.5 embryonic hippocampus in MEM with B27 supplement and 5% FCS and plated onto glass coverslips coated with poly- L -lysine. Two days after plating, 10 μM ara-C was added to prevent glial cell proliferation. For DiI labelling of culture neurons, cells were fixed in 2% paraformaldehyde in PBS for 4 h at room temperature. During the fixation, DiI (Molecular Probes) was loaded on the soma of GFP-positive neurons. After fixation, cells were washed three times with PBS. We analysed fixed numbers of spines (50 per each neurons) that were selected automatically using random numbers. Immunostaining of dissociated neurons and brain sections Hippocampal neuronal cultures were fixed in 2% paraformaldehyde. For immunocytochemistry of AMPA and NMDA receptors, cells were fixed with methanol solution at −20 °C. For immunostaining of the brain sections, mice were anesthetized with a lethal dose of barbiturate and perfused with 4% paraformaldehyde. The brains were dissected and cut into 40-μm thick slices using a vibratome. Both culture preparations and brain sections were treated with 0.2% Triton X-100 in PBS, blocked with 5% NGS (or normal donkey serum) and then reacted with the primary antibodies, followed by the secondary antibodies. Images were obtained by using a Fluoview-1000 confocal laser-scanning microscope (Olympus) with either a X10 dry lens (Olympus, UPlanApo, numerical aperture (NA (numerical aperture)) 0.40), a X20 dry lens (Olympus, UPlanApo, NA 0.7) or a X60 oil-immersion lens (Olympus, PlanApoN, NA 1.42). Image analyses Image analyses and quantification were performed by using Metamorph or ImageJ software. To determine the intensity of PSD proteins, we utilized two-dimensional object segmentation by fast Fourier transform of anti-PSD-95 or anti-Homer fluorescence spots. Images were processed with a high-pass filter to isolate objects, with the sizes comparable to single PSD clusters. The next steps of image analyses were as described previously [49] . For spinophilin cluster isolation, fast Fourier transform and the ensuing thresholding of the images could not be applied, mainly because of the heterogeneity of spinophilin distribution. To accurately measure the intensity of spinophilin in the spines, fluorescence intensity of the dendritic shafts was first subtracted from the original fluorescence images. The subsequent steps were identical to the measuring processes for PSD proteins. To perform Sholl analysis, dendrite morphology was tracked by Neuron J [50] and the data were quantified using the Sholl Analysis plugin for ImageJ software. Dendritic protrusions with their widths larger than half of their lengths were classified as mushroom spines. The other spines were classified as thin spines [20] . We performed blind analysis of images in several key experiments. The data confirmed by blind analyses of multiple experimenters include Fig. 2c , d , 3d . Time-lapse imaging of dissociated hippocampal neurons Live cells in the culture medium were mounted in a chamber at 37 °C with constant flow of air containing 5% CO 2 . Images were obtained on a Fluoview-1000 confocal laser-scanning microscope (Olympus) with a X60 oil-immersion lens (Olympus, PlanApoN, NA 1.42) at an additional electric zoom factor of 1–2.5 × . Multiple optical sections (z-spacing of 0.3–0.4 μm) were acquired and recombined using a maximum brightness operation. Electrophysiology mEPSCs and evoked EPSCs were recorded from neurons at 16 DIV at room temperature in the voltage-clamp configuration. The extracellular solution contain the following (in mM): 119 NaCl, 2.5 KCl, 25 HEPES, 30 D-glucose, 2 CaCl 2 and 2 MgCl 2 , pH 7.4. mEPSCs were recorded in the presence of 1 μM tetrodotoxin, 1 μM strychnine, 10 μM bicuculline and 10 μM glycine. Neurons were voltage clamped at −70 mV. mEPSCs were analysed using Clampfit 9.2 and MiniAnalysis program 6.0.3. For most experiments, only cells with 70–100 events were included in the analysis. Evoked EPSCs were recorded in the presence of 1 μM strychnine, 10 μM bicuculline and 10 μM glycine. Synaptic responses were evoked by electrical stimulation with a glass electrode filled with 1 M NaCl. AMPA receptor- and NMDA receptor-mediated EPSCs were obtained by evoking dual component responses while voltage-clamping neurons at −70 mV. A volume of 10 μM CNQX was then added to obtain the pure NMDA receptor-mediated EPSC at +40 mV, and the AMPA receptor component was derived by subtracting the NMDA receptor EPSC from the compound EPSC at −70 mV. Electrodes were filled with solution containing the following (in mM); 156 Cs-methanesulfonate, 6 KCl, 1.2 CaCl 2 , 2.4 MgCl 2 , 12 HEPES, 13.2 EGTA, 4 Mg-ATP, 1.5 Na-GTP and 5 QX-314, pH 7.4. All potentials were corrected for the liquid junction potential (9 mV). Recordings were performed with the MultiClamp 700B amplifier (Axon Instruments, Foster City, CA, USA). Records were filtered at 1–2 kHz and acquired at 10 kHz. Series resistance values were <20 MΩ. Evoked EPSCs were analysed using Clampfit 9.2 and Origin 8.0. Golgi–Cox impregnation See Supplementary Methods . PASME Design and properties of pThy1-S-ER T2 CreER T2 and β-actin promoter-FloxedStop-GFP plasmids were as described previously [21] . We introduced four types of plasmids (pThy1-S-ER T2 CreER T2 , β-actin promoter-FloxedStop-GFP, β-actin promoter-RFP and the DCLK1 shRNA plasmid) together by using in utero electroporation at E14 or E15 (ref. 51 ). In utero electroporation into the hippocampal neurons was performed at E15 as described previously [52] . Cre recombinase activity was induced by injecting 4-hydroxytamoxifen three times at postnatal days 14–16. The Thy1-S promoter, a short variant of the Thy1 promoter, supports expression of the downstream gene ubiquitously in immature neural precursors, but highly selective expression in the postnatal neocortex. Therefore, postnatal induction of ER T2 CreER T2 activity by 4-hydroxytamoxifen injection results in excision of FloxedStop sequences from the GFP reporter plasmids only in a small subset of differentiated pyramidal neurons. At postnatal days 21–23, mice were perfused with 4% paraformaldehyde; the brains were dissected and cut into 100-μm thick sections using a vibratome. The sections were stained with anti-GFP and anti-DsRed2 antibodies, followed by Alexa488- or Cy3-conjugated secondary antibodies. How to cite this article: Shin, E. et al. Doublecortin-like kinase enhances dendritic remodelling and negatively regulates synapse maturation. Nat. Commun. 4:1440 doi: 10.1038/ncomms2443 (2013).